Organic magnetoelectroluminescence for room temperature transduction between magnetic and optical information Magnetic and spin-based technologies for data storage and processing provide unique challenges for information transduction to light because of magnetic metals’ optical loss, and the inefficiency and resistivity of semiconductor spin-based emitters at room temperature. Transduction between magnetic and optical information in typical organic semiconductors poses additional challenges, as the spin–orbit interaction is weak and spin injection from magnetic electrodes has been limited to low temperature and low polarization efficiency. Here we demonstrate room temperature information transduction between a magnet and an organic light-emitting diode that does not require electrical current, based on control via the magnet’s remanent field of the exciton recombination process in the organic semiconductor. This demonstration is explained quantitatively within a theory of spin-dependent exciton recombination in the organic semiconductor, driven primarily by gradients in the remanent fringe fields of a few nanometre-thick magnetic film. Organic semiconductor devices have become a ubiquitous lighting technology owing to their flexibility, inexpensive character and highly efficient light output. Organic information processing also occupies an important niche, where computational speed is less important than flexibility or expense. Organic semiconductor sandwich devices, used for example in organic light-emitting diodes (OLEDs), consist of a thin film of an organic semiconductor (or several layers thereof) sandwiched between a bottom and top electrode. The organic semiconductor is typically intrinsic, and is essentially void of charge carriers. Therefore one of the electrodes is chosen to efficiently inject electrons, and the other to efficiently inject holes. For this purpose low and high work function metals, respectively, are chosen. Recombination of these electron-hole pairs leads to electroluminescence (EL) in the OLED. Nonvolatile information storage in organic electronics poses a challenge, as organic semiconductor flash memory currently has high leakage currents owing to the large electric fields required to change the transport properties of organic semiconductors [1] . The non-volatility, speed, and low energy consumption of the magnetic memory make it fundamentally attractive for integration with organics. Typical approaches for integrating optical and magnetic devices rely on magneto-optical effects, which require a strong spin–orbit interaction that most organic materials lack [2] , [3] . Use of spin injection provides a way to control the optical emission of an OLED, taking advantage of a spin-dependent exciton recombination process [4] , [5] , [6] , although magnetic metals have large impedance mismatches with organics. This impedance mismatch can be overcome using coupling through a magnet’s fringe field at zero applied field (remanent field) as demonstrated in organic electronic devices [7] , [8] , [9] . Efficient coupling via the magnet’s remanent field between light emission in organic devices and a magnetic memory would broaden the range of applicability of flexible, inexpensive organic electronics. External magnetic field effects on the conductivity and luminescence of an organic film are already known. Transport of the injected carriers through the organic film occurs via a sequence of hops along a path connecting the top electrode to the bottom electrode, and the rate of transport and/or recombination is markedly affected by variations in the local magnetic field along the path, as found in numerous experimental and theoretical studies [10] , [11] , [12] , [13] , [14] , [15] . In the transport regime, this effect is known as organic magnetoresistance (OMAR), and for light emission it is denoted as organic magnetoelectroluminescence (OMEL). Typically the source of the inhomogeneous field is the nuclear hyperfine field, which is random and spatially uncorrelated. The origin of OMAR can be traced back to interactions between paramagnetic charge pairs that occur at bottle-neck sites (sites that crucially affect the transport and/or electroluminescent properties). These interactions are often spin selective, and the reaction rate depends on the angle between the local spin-quantization axis (provided by the local magnetic field) for the two paramagnetic species. An applied magnetic field exceeding the hyperfine field strength forces this angle to be close to zero everywhere in the film, which shows up as magnetoconductance (MC) or magnetoelectroluminescence (MEL). The exact nature of the paramagnetic pairs remains hotly debated, and the possibilities include electron-hole pair recombination to form singlet or triplet excitons [12] , e – e or h – h recombination to form singlet bipolarons [13] and collision reactions between electrons or holes with long lived triplet excitons [14] . Here, we report that the fringe field resulting from a magnetic film a few nanometres thick can be used to control the electroluminescent output of an OLED at room temperature. Large gradients in the magnitude of the random local field lead to fringe-field-driven MC and MEL, and devices were constructed that utilize fringe fields from an unsaturated magnetic film to supply such gradients [7] , [8] , [9] . Electrically insulated magnetic films prove that fringe fields, and not electrical currents, are responsible for the coupling between the ferromagnetic layer and the OMAR/OLED device. This paper primarily discusses such fringe-field effects, but ‘ordinary’ OMAR and OMEL (based on, for example, hyperfine fields) are also investigated as a reference. As the fringe-field MEL mechanism is driven by fringe-field gradients, independent of the mechanism of ordinary OMAR and OMEL, the effects presented here should be found in organic materials independent of the mechanism of OMAR and OMEL, including in materials where there is no OMAR and OMEL [9] . We further simulate the effects of fringe-field gradients on the spin-dependent exciton recombination in the OLED, based on a simple model of the fringe-field gradients, and find excellent quantitative agreement with the measurements. These results provide a concrete demonstration of the potential for transduction between magnetic and optical information using fringe-field effects on OLED emission. Magnetic fringe-field effects on MC and MEL Our devices are OMAR/OLED devices fabricated on top of a ferromagnetic thin film, as shown in Fig. 1a . The device fabrication starts with the metal deposition of a ferromagnetic multilayered thin film made of Cobalt (Co) and Platinum (Pt). Those films have perpendicular magnetic anisotropy; the spins tend to align in the direction orthogonal to the film plane. In presence of a large magnetic field out of the film plane, the Co|Pt films are uniformly magnetized with all the spins pointing opposite to the direction of the applied field. At lower fields, the films form magnetic domains—some regions with spins pointing up and others with spins pointing down—to lower the magnetostatic energy. These magnetic domains create strong, spatially varying fringe fields close to the surface of the Co|Pt films, which penetrate the OMAR/OLED device. In order to electrically insulate the OMAR/OLED device from the ferromagnetic film, we deposit a thin dielectric followed by a conductive non-magnetic layer on top of the magnetic film. However, the strength and spatial correlation length of magnetic fringe fields depend sensitively on the distance from the magnetic film to the organic film. The insulating layer increases this distance reducing the effect. As a result, we report results primarily on devices without this layer, which show the largest effects, and study devices with insulating layers to rule out spin injection and tunnelling anisotropic magnetoresistive effects. 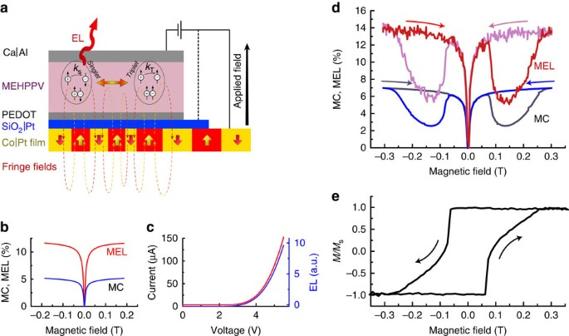Figure 1: Magnetoconductance (MC) and magnetoelectroluminescence (MEL) in organic semiconductor devices. (a) Schematic of the device structure used for fringe-field MC and MEL measurements. The device consists of a standard OMAR/OLED device fabricated on top of a ferromagnetic film, which need not be in electrical contact with the organic device. A SiO2layer was used in some devices to electrically isolate the magnetic film from the organic device. The electroluminescence (EL) is collected through the semitransparent top contact. (b) MC and MEL responses to an external magnetic field of a reference OMAR/OLED device without the magnetic film and (c) IV and EL versus voltage for the reference device. (d) MC and MEL responses of the complete organic fringe-field device. (e) MagnetizationMrelative to the saturation magnitizationMSof the ferromagnetic film as obtained by MOKE. All data are for room temperature. Figure 1: Magnetoconductance (MC) and magnetoelectroluminescence (MEL) in organic semiconductor devices. ( a ) Schematic of the device structure used for fringe-field MC and MEL measurements. The device consists of a standard OMAR/OLED device fabricated on top of a ferromagnetic film, which need not be in electrical contact with the organic device. A SiO 2 layer was used in some devices to electrically isolate the magnetic film from the organic device. The electroluminescence (EL) is collected through the semitransparent top contact. ( b ) MC and MEL responses to an external magnetic field of a reference OMAR/OLED device without the magnetic film and ( c ) IV and EL versus voltage for the reference device. ( d ) MC and MEL responses of the complete organic fringe-field device. ( e ) Magnetization M relative to the saturation magnitization M S of the ferromagnetic film as obtained by MOKE. All data are for room temperature. Full size image A conducting polymer layer (20 nm) of poly(3,4-ethylenedioxythiophene) poly(styrenesulphonate) (PEDOT:PSS, referred to as simply PEDOT from now on) was spin-coated from water suspension and serves as the hole-injecting layer. PEDOT is commonly employed for this purpose in OLED devices [16] . We chose poly(2-methoxy-5-(2-ethylhexyloxy)-1,4-phenylenevinylene) (MEHPPV) as the luminescent polymer, as it is widely used as a red emitter in OLEDs [17] . The MEHPPV layer (55 nm) was deposited by spin coating from toluene solution. Finally, calcium (Ca) (6 nm, serving as the electron-injecting top contact) covered by aluminium (Al) (12 nm) was deposited by vacuum evaporation through a shadow mask. The active device area is roughly 1 mm 2 . The Al-capping layer is required to protect the highly reactive Ca layer. The contributions of the PEDOT and Ca electrodes to the device resistance (and magnetoresistance (MR)) are negligible, as they are metals, whereas MEHPPV is an intrinsic semiconductor. The EL is measured through the semitransparent top electrode, and recorded by a photomultiplier tube. All measurements reported here are at room temperature. Figure 1b shows a typical MC and MEL trace, and Fig. 1c the current-voltage (IV) and EL curves, for an organic device without a magnetic film and whose MC/MEL is therefore caused by the random hyperfine fields, as described above. This device will serve as a reference when, later on, we will discuss fringe-field-induced MC/MEL. It is seen that the hyperfine-induced MC and MEL responses have a magnitude of ≈5% and ≈10%, respectively, in our MEHPPV devices. The effects essentially saturate for applied fields in excess of 0.1 T, are non-hysteretic and have a full width at half maximum of ~20 mT. The effects are also independent of the direction of the applied magnetic field, and nearly independent of the MEHPPV layer thickness. In the present work, we have chosen to work with a thin MEHPPV layer (55 nm) such that the distance from the ferromagnetic film does not vary much between different locations in the MEHPPV film. Now we turn our attention to the MC/MEL responses of the fringe-field OMAR devices, and the correlation between these effects and the film magnetization, M . Figure 1d shows the measured MC and MEL curves, and Fig. 1e shows the magnetization loop measured by magneto-optic Kerr effect (MOKE) (see Methods section). In these measurements, the magnetic field is applied perpendicularly to the device plane, and is swept smoothly from large negative to large positive fields and back (black lines). It is seen that the magnetization response is hysteretic, and that M assumes its saturation value M S for fields larger than ~0.25 T in magnitude. M is unsaturated between roughly 0.05 and 0.25 T. The MC/MEL curves outside the unsaturated magnetization regime clearly mirror the data in non-magnetic devices (panel b), and are explained by the ‘normal’ hyperfine OMAR effect. In the unsaturated region, the data curves develop characteristic ‘ears’. These are the signature of fringe-field effects. We have previously given a detailed experimental and theoretical characterization of the transport aspect of this effect [7] , [8] , [9] . In the present work, we demonstrate for the first time that fringe-field effects lead to a sizable room temperature MEL response, of up to 6% at room temperature for the present device. This can be comparable to MEL effects that occur only at low temperature, such as those recently reported in spin-valves [6] and high magnetic field effects for OLEDs [18] . Next, we examine the relation between the magnetic film’s response characteristics and MC/MEL by fabricating OMAR/OLED devices on several different ferromagnetic electrodes. In this work, the different magnetic responses are studied by fabricating ferromagnetic films consisting of Cobalt (Co) and Platinum (Pt) multilayers with a different number of repeats, n . We studied devices with n =5, 10, 20 and 30 (film thicknesses varied from 4 to 24 nm). The magnetization in the ferromagnetic films reverses through nucleation, growth and annihilation of magnetic domains. When the magnetic films are saturated (all spins pointing towards the same direction) there are no magnetic fringe fields on top. When the magnetic films are unsaturated the strength of the magnetic fringe fields created by magnetic domains increases (almost linearly) with the thickness of the ferromagnetic layer (that is, with the number of repeats). Properties of Co|Pt ferromagnetic films have been characterized in detail (see refs 7 , 8 ). The data in Fig. 2 shows that the hysteretic MR of the organic layer is directly correlated with the hysteretic magnetization of the ferromagnetic film. The fringe-field ‘ears’ occur only in the unsaturated regime, where the film’s magnetization breaks into domains with fringe fields occurring near the domain boundaries. 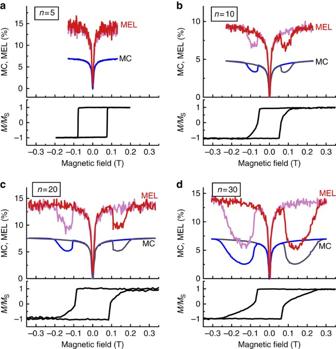Figure 2: Correlation between MC/MEL and magnetization for several different ferromagnetic films. (a–d) MC and MEL responses of organic fringe-field devices using different ferromagnetic films. The magnetic films are Co|Pt multilayers with a different number of Co|Pt repeats,n, resulting in different magnetization loops as evidenced by the MOKEM/MS. In all cases (a–d) the fringe-field response correlates exactly with the field range where the magnetic film is unsaturated, and therefore emits fringe fields into the organic device. Figure 2: Correlation between MC/MEL and magnetization for several different ferromagnetic films. ( a – d ) MC and MEL responses of organic fringe-field devices using different ferromagnetic films. The magnetic films are Co|Pt multilayers with a different number of Co|Pt repeats, n , resulting in different magnetization loops as evidenced by the MOKE M / M S . In all cases ( a – d ) the fringe-field response correlates exactly with the field range where the magnetic film is unsaturated, and therefore emits fringe fields into the organic device. 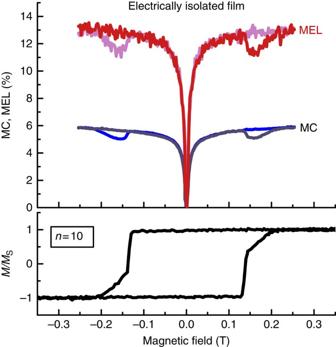Figure 3: Demonstration that the fringe-field effect is a result of magnetic, rather than electrical coupling. MC and MEL responses of an organic fringe-field device where the magnetic film is electrically isolated from the organic device by insertion of a SiO2layer between them. This control experiment is important for establishing the correct interpretation of the data (see text), but results in a greater distance between magnetic film and organic device, leading to a smaller coupling between the two and a smaller fringe-field effect. Full size image Studies with electrically isolated magnetic films Figure 3 shows data similar to that reported in Fig. 2 , but now for a device with an additional SiO 2 layer inserted between the magnetic film and the OMAR/OLED device. These data exhibit all the same characteristics of the data without the insulating layer, and prove that the coupling between the magnetic film and the organic device is magnetic rather than electrical in nature. In particular this excludes mechanisms such as tunnelling anisotropic MR and spin-injection effects as the origin of the observed effects. The ‘ears’ are, however, significantly smaller in magnitude. This was to be expected, because the insulating layer leads to a significantly larger separation between the magnetic film and OMAR/OLED device as the overall spacer layer thickness increases from 20 to 45 nm with the layer inserted. We have previously examined [8] the dependence of the magnitude of the fringe-field MR on the spacer layer thickness. Figure 3: Demonstration that the fringe-field effect is a result of magnetic, rather than electrical coupling. MC and MEL responses of an organic fringe-field device where the magnetic film is electrically isolated from the organic device by insertion of a SiO 2 layer between them. This control experiment is important for establishing the correct interpretation of the data (see text), but results in a greater distance between magnetic film and organic device, leading to a smaller coupling between the two and a smaller fringe-field effect. Full size image Control of EL with remanent fields Magnetic domains can be present at zero applied field in our magnetic films. Such remanent states are prepared by applying a perpendicular field close to the film’s coercive field and then removing it (see Fig. 4a ). Magnetization measurements and imaging prove that remanent domain states relax only slightly on removal of the field. Therefore, we have access to remanent magnetization states ranging from negative to positive saturation. At zero applied field, we observed how remanent fringe fields increase the conductance of the organic layer MEHPPV, suppressing OMAR. The same effect with a smaller strength was observed in the organic semiconductor Alq 3 (ref. 8 ). 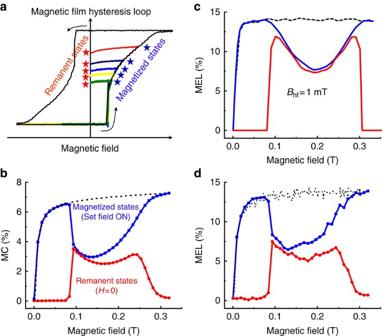Figure 4: Correlation between a remanent magnetic state of the magnetic film and the MC/MEL. In these measurements the applied magnetic field plays an auxiliary role, and is used to write (‘set’) a particular remanent magnetic state, corresponding to a particular domain configuration and particular fringe-field pattern, and to erase (‘reset’) this configuration by replacing it with a saturated state without domains. This saturated state without domains is also used as the reference state against which we measure the MC and MEL percentage responses. Referring to the magnetization loop of an example magnetic film, (a) shows the procedure to set and reset different remanent states. The set field (blue star) is used to select a magnetic state. As the set field is being removed, the film remains in essentially the same state as evidenced by the only small amount of relaxation in magnetization between the write state (blue star) and remanent state (red star). (b) Conductance and (d) electroluminescence referenced to a fully saturated state measured in different magnetic states of the ferromagnetic film vs set field strength (red curve). For comparison, the conductance and electroluminescence value measured while the set field is still on is also shown (blue curve). Grey dashed curves correspond to measured values of conductance (b) and electroluminescence (d) at the set field when the magnetic film is saturated (blue and purple curves inFig. 2). (c) Theoretical calculation following text, using switching fields fromFig. 1e, to be compared withd. Grey dashed curve is calculation with fringe fields absent. Figure 4b,d shows MC and MEL of a 55-nm-thick MEHPPV film on top of a magnetic layer both in presence of and at zero magnetic field. The blue line depicts the measured values in presence of magnetic field, whereas the red lines trace the values measured after removing the applied field (a sketch of the measuring sequence is shown in Fig. 4a ). We first saturated the sample with a large negative field, then we set a positive field value from 0 to 0.3 T and measured the conductivity of the organic layer (blue points) and then we removed the applied field and again measured the organic’s conductivity (red points). Here we show that the electroluminiscence increases up to 6% for remanent magnetic domain states of the ferromagnetic layer. In contrast to fringe fields from the same domain configuration in an applied magnetic field (near the coercive field), the MEL increases rather than decreases. Figure 4: Correlation between a remanent magnetic state of the magnetic film and the MC/MEL. In these measurements the applied magnetic field plays an auxiliary role, and is used to write (‘set’) a particular remanent magnetic state, corresponding to a particular domain configuration and particular fringe-field pattern, and to erase (‘reset’) this configuration by replacing it with a saturated state without domains. This saturated state without domains is also used as the reference state against which we measure the MC and MEL percentage responses. Referring to the magnetization loop of an example magnetic film, ( a ) shows the procedure to set and reset different remanent states. The set field (blue star) is used to select a magnetic state. As the set field is being removed, the film remains in essentially the same state as evidenced by the only small amount of relaxation in magnetization between the write state (blue star) and remanent state (red star). ( b ) Conductance and ( d ) electroluminescence referenced to a fully saturated state measured in different magnetic states of the ferromagnetic film vs set field strength (red curve). For comparison, the conductance and electroluminescence value measured while the set field is still on is also shown (blue curve). Grey dashed curves correspond to measured values of conductance ( b ) and electroluminescence ( d ) at the set field when the magnetic film is saturated (blue and purple curves in Fig. 2 ). ( c ) Theoretical calculation following text, using switching fields from Fig. 1e , to be compared with d . Grey dashed curve is calculation with fringe fields absent. Full size image Theory of magnetic fringe-field effects on MC and MEL We now examine whether the large fringe-field effects observed in the MEL can be explained by theory. We consider a two-site model where an electron and hole (a polaron pair) occupy two nearby sites. The spin configuration of the polaron pair undergoes transitions due to the different magnetic interactions present; in our case these interactions consist of which are the applied, hyperfine and fringe-field Hamiltonians, respectively. The polaron pairs recombine into excitons at different rates, k S and k T , depending on the pair’s spin, as the singlet and triplet states have different energies and wavefunctions [19] (see schematic Fig. 1a ); alternatively the pair could disassociate at a rate k D . Once an exciton is formed, the large exchange energy precludes any further spin evolution. In the absence of large spin–orbit interactions, spin selection rules dictate that exciton recombination (that is, photon emission) occurs only from the singlet exciton state. Assuming that radiative recombination is the only viable pathway for a newly formed singlet exciton, each singlet exciton will produce a single photon such that MEL can be defined in terms of X S , the singlet fraction of excitons: [ X S ( B 0 )− X S (0)]/ X S (0). To calculate the MEL, we employ the stochastic Liouville equation for the polaron pair spin density matrix, ρ [20] , [21] : where P S and P T are the singlet and triplet projection operators. The steady-state singlet and triplet exciton fractions are [22] where i runs over S and T . All rates (times) are in units of the hyperfine field frequency (period), γ e B hf (1/γ e B hf ) where B hf is the width of the Gaussian distribution of hyperfine fields. For simplicity we assume γ e = γ h and k D =0. To proceed with the calculation, one must have knowledge of the fringe fields present in the organic layer. In our previous analysis [9] on fringe-field-induced magnetoresistance, elementary magnetostatics were used to calculate fringe fields from X-ray magnetic circular dichroism (XMCD) images of the magnetic domains. The samples described herein have the same composition. We use therefore the statistical analysis from the aforementioned XMCD images to model the fringe-field distributions. Given the fact that fringe fields vanish at magnetic saturation and are largest and most varying at M =0, we model the fringe-field distribution as a normal distribution with mean zero and a field dependent standard deviation. Each component of the fringe-field ( B ff ) gradient, G ff , is modelled likewise. The field dependent standard deviations follow a parabola defined in the upper half-plane according to where B L is the field at which the magnet starts developing domains (obtainable from either the MOKE data or the MEL measurements) and B C is the field corresponding roughly to M =0. and mark the parabola's vertex and are the only free parameters. However, from analysis of samples of the same composition on which XMCD images have been acquired, their values are roughly 40 mT and 1 mT nm −1 , respectively, for a spacer width of 20 nm. The results of this theory and model are shown in Fig. 4c . The B L and B C are chosen from Fig. 1e . The values of k S (=1.5 γ e B hf ) and k T (=5 γ e B hf ) are chosen to achieve a saturated MEL percentage near that of Fig. 1d , ~14%. The values for the hopping rates fall into an intermediate hopping regime ( k s ~γ e B hf ) that produces a fringe-field effect. Remanent fringe fields generated from the domain structure of the magnetic film cause the observed marked modification of the EL from an OLED at room temperature. As a uniform, perpendicularly magnetized film produces no remanent fields, the source of these fringe fields is the region where the magnetization changes most rapidly, corresponding to domain walls. The faster the magnetization changes, or the smaller the domain size, the larger the remanent fields. Thus this approach of interfacing magnetic information encoded in the domain structure with an OLED should become more effective and efficient as the magnetic domain sizes shrink. We note as well that the MEL is significantly larger than the MC, indicating that (for MEHPPV) fringe-field optical coupling and readout will have greater sensitivity than fringe-field electrical coupling and readout of magnetic information. Fringe-field device fabrication The organic semiconductor semispin valve consists of a ferromagnetic layer, a hole-injecting layer, an organic semiconductor and a top electrode. The ferromagnetic electrode is a Co|Pt multilayer with the number of repeats varying from 5 to 30 deposited using electron-beam evaporation in ultra high vacuum on oxidized Si wafers for device studies, and Si supported Si 3 N 4 membranes for magnetic domain-imaging studies using an X-ray transmission microscope. Optical lithography is used to define lines in the ferromagnetic thin film. A hole-injecting layer, conducting polymer PEDOT:PSS, was deposited by spin coating from an aqueous suspension (suspension purchased from H. C. Starck, CLEVIO P VP AI 4083). A 55-nm-thick film of organic semiconductor MEHPPV (purchased from American Dye Source, Inc.) was deposited by spin coating with 3 mg ml −1 solution in toluene. The electron-injecting layer, Ca (6 nm) covered by Al (12 nm) was deposited by thermal evaporation at room temperature through a metal stencil to obtain a cross-point device geometry. The ferromagnetic electrodes were characterized by magnetic force microscopy, ferromagnetic resonance, vibrating sample magnetometery and MOKE. Measurements MR measurements were done in a closed-cycle He cryostat positioned between the poles of an electromagnet. The measurements reported here are all at room temperature. MR measurements were performed using a Keithley 2400 sourcemeter. EL was measured using a photomultiplier tube through the top electrode Ca/Al. X-ray measurements were performed at the Advanced Light Source at the Lawrence Berkeley National Laboratory. Images were taken with a XM-1 zone-plate microscope at beamline 6.1.2. How to cite this article: Macià, F. et al. Organic magnetoelectroluminescence for room temperature transduction between magnetic and optical information. Nat. Commun. 5:3609 doi: 10.1038/ncomms4609 (2014).